Bicc1 and Dicer regulate left-right patterning through post-transcriptional control of the Nodal inhibitor Dand5 Rotating cilia at the vertebrate left-right organizer (LRO) generate an asymmetric leftward flow, which is sensed by cells at the left LRO margin. Ciliary activity of the calcium channel Pkd2 is crucial for flow sensing. How this flow signal is further processed and relayed to the laterality-determining Nodal cascade in the left lateral plate mesoderm (LPM) is largely unknown. We previously showed that flow down-regulates mRNA expression of the Nodal inhibitor Dand5 in left sensory cells. De-repression of the co-expressed Nodal, complexed with the TGFß growth factor Gdf3, drives LPM Nodal cascade induction. Here, we show that post-transcriptional repression of dand5 is a central process in symmetry breaking of Xenopus , zebrafish and mouse. The RNA binding protein Bicc1 was identified as a post-transcriptional regulator of dand5 and gdf3 via their 3′-UTRs. Two distinct Bicc1 functions on dand5 mRNA were observed at pre- and post-flow stages, affecting mRNA stability or flow induced translational inhibition, respectively. To repress dand5 , Bicc1 co-operates with Dicer1, placing both proteins in the process of flow sensing. Intriguingly, Bicc1 mediated translational repression of a dand5 3′-UTR mRNA reporter was responsive to pkd2 , suggesting that a flow induced Pkd2 signal triggers Bicc1 mediated dand5 inhibition during symmetry breakage. The Nodal signaling cascade is central in setting up organ situs during embryonic development [1] , [2] . In Xenopus , the Tgfβ ligand Nodal1 is activated in the LPM of the neurula embryo, where it induces its own transcription, that of its feedback inhibitor lefty and the homeobox transcription factor pitx2 . Cilia are required for Nodal cascade induction [3] , [4] , [5] in fish, amphibian and mammalian embryos, but not in reptiles and birds [1] , [6] , [7] . The archenteron (primitive gut or remnants thereof) transiently harbors the ciliated epithelium of the left-right organizer (LRO) during neurula stages. In frogs, the gastrocoel roof plate (GRP [8] ) develops from precursor cells, i.e., superficial mesoderm, which is specified during the early gastrula stages. GRP cells have different fates, which correlate with specific properties. They are notochordal (cLRO) at the midline or somitic (sLRO) more laterally. The GRP, like other vertebrate LROs, is typically characterized by motile cilia at its center and immotile, supposedly sensory cilia at its lateral borders [5] . The posterior orientation and tilt of motile cilia, and their intrinsic clockwise rotation, give rise to a leftward fluid flow in the extracellular space that is sensed at the left LRO margin by a ciliary complex containing the ion-channel Pkd2 (TRPP2/Polycystin2). It is generally believed that the cation channel Pkd2, which we initially characterized as an LR determinant in a pkd2 knockout mouse [9] , is central to flow sensing. In mice and fish, left-asymmetric calcium spikes in lateral LRO cells were reported, which were depending on a ciliary Pkd2 function. Calcium influx, therefore, seems to represent the initial response to flow sensing [10] , [11] . The decisive molecular target of leftward flow is the repression of the Nodal inhibitor dand5 (former coco in frog; Cerl2 in mouse; charon in fish) at the left LRO margin [12] , [13] , [14] . nodal is co-expressed with dand5 in time and/or space and thereby inhibition of Dand5 protein synthesis results in de-repression of Nodal signaling. As a consequence, Nodal bound to the Gdf3 protein (former derriére in frog; Gdf1 in mouse) is transferred to the left LPM, where it induces the left-asymmetric Nodal signaling cascade [15] , [16] . A critical component of LR patterning is the flow-dependent repression of Dand5, manifested partially by a left-sided reduction of dand5 mRNA in vertebrate embryos. In mice, dand5 mRNA is destabilized via its 3′-UTR in a flow-dependent manner [13] . However, the timing of dand5 asymmetry raises the possibility that post-transcriptional mRNA decay might be insufficient for reducing Dand5 protein levels and suggests that additional mechanisms contribute to repression. In frog, dand5 mRNA asymmetry is most pronounced at late neurula, i.e., the very stages (st. 19–21) in which nodal1 is already expressed in the left LPM [12] . In addition, left-sided dand5 mRNA decay in Xenopus is observed in a maximum of ~80% of wt specimens, whereas left Nodal cascade induction and the arrangement of inner organs were undisturbed in 95% of cases. Thus, the frequency of dand5 asymmetry is insufficient to explain the robust occurrence of wildtype organ asymmetry (situs solitus). The data indicates that detectable dand5 mRNA asymmetry occurs too late and infrequently to be functionally relevant and suggests that flow-dependent dand5 repression might also include translational inhibition. A protein that could exert both proposed post-transcriptional functions is Bicc1 (BicC family RNA-binding protein 1). Bicc1 binds to selected mRNAs and modifies translation post-transcriptionally, in a positive [17] or negative context-dependent manner [18] , [19] . Further, Bicc1 localizes to P-bodies, cytoplasmic complexes involved in mRNA stability and turnover [17] , [20] , [21] . Interestingly, Bicc1 interacts with microRNAs (miRs), which function in post-transcriptional regulation of mRNA translation and integrity [22] . Previous studies indicated Bicc1 functions are important for LR patterning. bicc1 in frogs and mice is expressed in the LRO. bicc1 loss-of-function (LoF) impacts Wnt/planar cell polarity (PCP) signaling, resulting in unpolarized LRO cilia and perturbed leftward flow [20] . However, bicc1 expression in the frog LRO revealed strong enrichment of mRNA in nodal1 and dand5 positive sLRO cells (cf. Figure 3 in ref. [20] ), indicative of a separate, specific function in these cells, which was not addressed at the time. 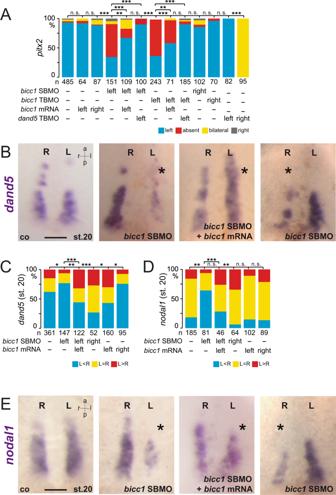Fig. 3: Bicc1-dependentdand5andnodal1expression in sLRO cells. AAbsence of left LPMpitx2expression inbicc1morphants, unilaterally injected on the left, was rescued by parallel knockdown ofdand5. Specificity of TBMO or SBMO was shown by co-injecting rescue mRNAs, i.e., mousebicc1orXenopus bicc1, respectively. Notedand5knockdown on the right efficiently inducedpitx2expression, as published.BLoss ofdand5mRNA at post-flow stages (st. 20) following left- and right-sidedbicc1SBMO injections. Controls (co) showed wt expression.dand5expression was restored by co-injectingbicc1rescue mRNA. Note enhanceddand5staining in rescued specimens.CQuantification ofdand5expression after knockdown ofbicc1. The effect was observed in the left and right sLRO cells.D,EDownregulation ofnodal1inbicc1morphants.DQuantification of results.EWt specimens show bilateralnodal1mRNA. Left or rightbicc1SBMO injections reducednodal1, which was restored by adding rescuebicc1mRNA. MO pmol/embryo:bicc1SBMO (L and S, each 1);bicc1TBMO, (L and S, each 1);dand5TPMO (0.5). Asterisks inBandEmark the injected side. Numbers (n) inA,C, andDrepresent analyzed specimens from more than three independent experiments. Statistical analyses were done with one-sided Pearson’s chi-square test, which was adjusted for multiple comparisons by Bonferroni (B) or Bonferroni–Holm (C,D). n.s. not significantp> 0.05; * significant,p< 0.05; ** highly significantp< 0.01; ***, very highly significantp< 0.001.pvalues and listing of individual experiments can be found in the source data file. st., stage. Scale bars inBandErepresent 100 µm. st. stage, a anterior, l left, r right, p posterior. Here, we show that the RNA-binding protein Bicc1 regulates dand5 mRNA stability and translation in LRO sensor cells. Approximately 139 nucleotides of the proximal dand5 3′-UTR are required and sufficient for Bicc1-mediated translational repression. Furthermore, within this small  sequence, we identify distinct sub-regions specific for dand5 mRNA stability and translational repression. In addition, we show that Bicc1 also regulates the translation of gdf3 , thereby influencing Nodal signaling directly. Finally, our data indicate that bicc1 functions together with dicer1 (the enzyme catalyzing the final step of miR biosynthesis) and pkd2 to mediate dand5 repression, and this function is evolutionary conserved in other organisms. Bicc1 represses dand5 translation Because of the allotetraploid genome of Xenopus laevis , 3′-UTRs of dand5 alloalleles were compared. Sequence conservation between S and L-alleles is low, except for the proximal 230 nucleotides downstream of the Stop-codon, which show 84% sequence identity (Supplementary Fig. 1A, B ). Asymmetric dand5 mRNA expression was found for both alleles, as visualized by in situ hybridization (ISH) of dorsal explants at stages 18 and 20 with antisense RNA probes specific for the 3′-UTRs of S- and L-alleles (Supplementary Fig. 1C, D ). Based on our previous identification of dand5 mRNA as a target of Bicc1 binding [18] we wondered whether Bicc1 regulates dand5 , the critical effector downstream of leftward flow [1] . To directly test this, an assay in animal cap explants was set up (AC assay; Fig. 1A ) which specifically analyzed Bicc1’s capacity to interfere with mRNA translation. We used mRNAs of our previously published dand5 .S 3′-UTR and newly cloned L 3′-UTR luciferase reporters (Supplementary Fig. 1B [18] ). Because bicc1 is not present in AC cells [23] , gain-of-function (GoF) experiments do not unravel any in vivo functions but reflect a somewhat artificial assay. dand5 mRNA, however, is maternally deposited at the animal pole [24] and thus post-transcriptional regulation might be active in AC cells. Injections were targeted to the animal region of the four-cell embryo and AC tissue was excised at the early gastrula stage 10 (Fig. 1A ). Reporter mRNAs harboring the full-length 3′-UTRs of the respective S and L-alleles of dand5 were translated, subsequently resulting in luciferase activity (Fig. 1B ). Co-injection of bicc1 mRNA, however, repressed luciferase activity of both reporters to ~20%. A full-length mouse bicc1 mRNA also repressed reporter activities, though less efficiently (Fig. 1B ). These experiments demonstrate a repressive effect of Bicc1 on a reporter protein expressed from an mRNA construct harboring the dand5 3′-UTR. Fig. 1: Bicc1 represses dand5 mRNA translation via its proximal 3′-UTR. A Schematic depiction of dand5 reporter assay. dand5 3′-UTR sequences fused to luciferase coding were injected either with or without bicc1 mRNA into the animal region of four-cell embryos. At st. 10, the animal cap region was excised and assayed for luciferase activity. Adapted from refs. [65] and [66] . B Animal cap reporter assay following injections of dand5 S- or L 3′-UTRs alone or together with Xenopus ( bicc1 ) or mouse Bicc1 ( mbicc1 ) effector mRNAs. Note that both alloalleles were equally repressed. Note also that mbicc1 was efficient as a repressor as well. C Luciferase reporter constructs harboring different regions of the dand5 (S-allele) 3′-UTR. D Repression of translation is mediated through a proximal 139 nucleotides (nt) sequence element in the dand5 3′-UTR. E Schematic depiction of medial and distal target protector MOs (m-tpMOs or d-tpMOs) binding to the minimal Bicc1 responsive element (Bicc1RE) in the dand5 3′-UTR (L or S). F m- and d-tpMOs (0.4 or 0.5 pmol/embryo, respectively) interact differently with the luciferase reporter expression. m-tpMO blocked and d-tpMO boosted luciferase activity. Co-injection of d-tpMOs prevented Bicc1-dependent repression of the full-length dand5 reporters (L and S) and further enhanced their expressivity. N in B , D , and F represents the number of independent experiments. A pool of 10 animal caps was analyzed per experiment and treatment. Results from reporter mRNAs alone served as reference and were set to 100% RLU. Relative values of single experiments are depicted as blue dots. Data of at least three experiments are presented as mean value (bar) ±standard deviation (error bar, SD). Statistical analyses were done with a one-sided Student’s t test for two independent means (Bonferroni corrected) using the values of at least three individual experiments. p values, values for individual experiments, the mean values, and standard deviations are found in the source data file. n.s. not significant p > 0.05; * significant, p < 0.05; ** highly significant p < 0.01; ***, very highly significant p < 0.001; RLU relative luciferase units; Luc luciferase . Full size image Next, we asked which sequences in the 3′-UTR were required for translational inhibition by Bicc1. To do so, different regions of the 1818 nucleotides of dand5 .S 3′-UTR were deleted (Fig. 1C ). Deleting the proximal 568 nucleotides abrogated the repressing effect of Bicc1 (Fig. 1D ). This proximal sequence alone enabled translational repression to ~30% of wt, i.e., slightly less than the full-length 3′-UTR. Further narrowing down to nucleotides 1–139 allowed repression at wt levels while deleting additional 26 nucleotides (construct 1–103) abolished translational inhibition, suggesting that nucleotides 103–139 could be particularly important. For validation, a cyclin B1 reporter was used as negative, and a tdgf1 ( cripto ) reporter as a positive control, as previously reported [18] . To test whether the proximal element of the dand5 3′-UTR was instrumental in mediating Bicc1-dependent translational repression, antisense target protector morpholino oligomers (tpMOs) were designed. tpMOs have been recently used to block specific sequences in UTRs, i.e., miRNA or protein-binding sites, to analyze post-transcriptional regulation [25] . We specifically targeted the distal 103–139 region (d-tpMO) and 5′ adjacent medial sequences (m-tpMO) of the identified minimal Bicc1 responsive 3′-UTR in S and L. The medial tpMOs were complementary to nucleotides 65–89 for the L and S alloalleles ( dand5 .L m-tpMO; dand5 .S m-tpMO). The distal tpMOs were complementary to nucleotides 91–116 of the L ( dand5 .L d-tpMO) and 107–132 of the S ( dand5 .S d-tpMO) alloallele (Fig. 1E ; Supplementary Fig. 1B ). m-tpMOs alone efficiently repressed reporter mRNA translation, suggesting that the blocked sequence is critical for general expressivity (Fig. 1F ). Co-injection of the d-tpMOs with the full-length 3′-UTR dand5 reporter and bicc1 mRNA prevented repression (Fig. 1F ). The reporter activity was about two- to threefold enhanced by d-tpMOs, as was the reporter activity upon co-injection with d-tpMO in the absence of bicc1 (Fig. 1F ). These data show that additional components restrict dand5 reporter activity through interaction with its 3′-UTR, suggesting that the endogenous dand5 mRNA is under post-transcriptional control independently of Bicc1. Taken together the reporter assays confirm the role of the proximal 3′-UTR dand5 sequences in Bicc1-dependent repression, which we, therefore, termed “Bicc1 responsive element” (Bicc1RE; Supplementary Fig. 1B ). Bicc1 responsive element is required for LR asymmetry To underscore the functional relevance of our AC assays, we examined the in vivo effect of tpMOs on LR asymmetry. Injections were performed in a unilateral manner at the 4–8 cell stage and thereby the effects on flow receiving, left or right sLRO cells were analyzed separately. Targeting m-tpMOs (L or S) to left sLRO cells did not change pitx2 asymmetry at tadpole stages, whereas on the right, m-tpMOs induced ectopic pitx2 expression in the right LPM (Fig. 2A , B). In contrast, right-sided injections of d-tpMOs (either L or S allele) had no effect, whereas left application prevented pitx2 induction in the left LPM in close to 50% of specimens (Fig. 2A , C), suggesting that Bicc1RE is also required for dand5 repression in vivo. Importantly, co-injection of dand5 translation blocking morpholino (TBMO) rescued asymmetric pitx2 induction (Fig. 2C ), emphasizing d-tpMO specificity. These results suggest that medial and distal sub-regions of the Bicc1RE in the dand5 3′-UTR mediate different aspects of dand5 post-transcriptional regulation and therefore both impact on LR asymmetry. Fig. 2: Bicc1 responsive element (Bicc1RE) of the dand5 3′-UTR is required for LR asymmetry. A Uninjected control (co), m-tpMO, or d-tpMO-injected embryos showed left, bilateral, or absent pitx2 expression, respectively. Lateral views (left and right) of embryos are presented. Arrowheads mark pitx2 -positive lateral plate mesoderm. B Quantification of pitx2 results of m-tpMO-treated specimens. C Quantification of pitx2 asymmetry by d-tpMO injections. Note administration of dand5 TPMO together with d-tpMOs restored wt pitx2 expression. D Diminished dand5 mRNA expression by left-sided and right-sided m-tpMO injections compared with control. E Quantification of dand5 expression at post-flow stages (st.20) following m-tpMO treatment. F Quantification of dand5 expression in pre-flow specimens injected with m-tpMO. G Wildtype dand5 repression in control (co) and left- or right-sided d-tpMO injected specimens. H Quantification of dand5 asymmetry. Note flow-induced dand5 mRNA decay was observed in controls and following d-tpMO application. I Quantification of dand5 staining of pre-flow specimens (st.16) following d-tpMO injections. MO pmol/embryo: m-tpMO (L or S, 0.8); d-tpMO (L or S, 1). Asterisks in D and G mark injected side. Scale bars in D and G represent 100 µm. Numbers (n) in B , C , E , F , H , and I represent analyzed specimens from more than three independent experiments. Statistical analyses were done with one-sided Pearson’s chi-square test, which was adjusted for multiple comparisons by Bonferroni ( B , C ) or Bonferroni–Holm ( E , F , H , I ). p values and listing of individual experiments can be found in the source data file. n.s. not significant p > 0.05; **highly significant p < 0.01; ***very highly significant p < 0.001; st. stage; a anterior; l left; r right; p posterior. Full size image We then analyzed dand5 expression patterns following tpMO treatment. dand5 mRNA expression at post-flow stages (st. 20) was considerably reduced by m-tpMO irrespective of whether the right or left sLRO lineage was targeted (Fig. 2D, E ). Sided dand5 downregulation by m-tpMO was in agreement with either ectopic pitx2 induction in the right LPM or its wildtype expression in left injected specimens. Importantly, loss of dand5 mRNA was already observed in pre-flow stages (Fig. 2F , Supplementary Fig. 2A ), indicating independence of flow. Toxic effects by m-tpMOs were excluded because targeted sLRO cells depicted wt nodal1 expression (Supplementary Fig. 2A ). Thus, we identified a medially localized sub-region in the Bicc1RE, likely required for dand5 mRNA stability. Intriguingly, left-sided d-tpMO injections did not alter flow-induced downregulation of dand5 mRNA (Fig. 2G, H ), although pitx2 asymmetry was lost. Irrespective of which side was targeted, the frequency of stronger right-sided dand5 signals compared with left sLRO (R>L) in post-flow stages did not differ between untreated controls and d-tpMO injected specimens (Fig. 2G, H ). In pre-flow embryos (st. 16) no changes in dand5 expression were observed either (Fig. 2I , Supplementary Fig. 2C ). nodal1 expression was also not altered, showing that d-tpMOs did not cause unspecific detrimental effects (Supplementary Fig. 2D ). Our results suggest that the distal sub-region conveys flow-dependent repression specifically via dand5 translation but does not impair mRNA decay. Bicc1 regulates dand5 and nodal1 expression at pre-flow stages To connect our observed tpMO effects on the dand5 Bicc1RE to Bicc1 function, we performed bicc1 LoF experiments. X. laevis offers precise targeting of sLRO cells by microinjection of the left or right C2-lineage [26] , [27] , [28] , whereas avoiding the flow-generating cLRO (Supplementary Fig. 3A ). This injection setup circumvents described defects in cilia polarization. To knockdown bicc1 , a previously published TBMO [20] was used as well as a designed splice-blocking MO (SBMO). In both cases, two MOs were used which specifically targeted the S- or L-allele, which are both expressed during embryogenesis and encode identical proteins [29] . Injecting either MO separately did not affect laterality (Supplementary Fig. 3B ). In morphants, in which the sLRO was targeted by co-injection of S- and L-MOs, the LRO morphology and cilia polarization in cLRO and sLRO cells was unaffected, demonstrating proper targeting (Supplementary Fig. 3C, C’, D ). pitx2 expression, however, was predominately absent in morphants injected unilaterally on the left side (Fig. 3A ; Supplementary Fig. 2E ). Right-sided bicc1 LoF had no effect on pitx2 expression. MO-specificity was demonstrated by co-injecting full-length bicc1 mRNA that was not targeted by either MO (mouse Bicc1 , mbicc1 , in case of TBMO, and Xenopus bicc1 in case of SBMO), which rescued pitx2 expression in a significant proportion of specimens (Fig. 3A ; Supplementary Fig. 3E ). In addition, splicing of bicc1 pre-mRNA was affected in SBMO-treated specimens, shown by RT-PCR (Supplementary Fig. 3F ). Interestingly, GoF alone did not affect pitx2 (Fig. 3A ), which indicates that an excess of Bicc1 was not interfering with flow sensing or subsequent processes. Both bicc1 MOs gave virtually identical results, fulfilling yet another criterion for the controlled use of MOs [30] . Importantly, parallel LoF of bicc1 and dand5 in left sLRO cells rescued pitx2 expression (Fig. 3A ), which fits a scenario where Bicc1 acts downstream of flow and upstream of flow-mediated dand5 repression. Fig. 3: Bicc1-dependent dand5 and nodal1 expression in sLRO cells. A Absence of left LPM pitx2 expression in bicc1 morphants, unilaterally injected on the left, was rescued by parallel knockdown of dand5 . Specificity of TBMO or SBMO was shown by co-injecting rescue mRNAs, i.e., mouse bicc1 or Xenopus bicc1 , respectively. Note dand5 knockdown on the right efficiently induced pitx2 expression, as published. B Loss of dand5 mRNA at post-flow stages (st. 20) following left- and right-sided bicc1 SBMO injections. Controls (co) showed wt expression. dand5 expression was restored by co-injecting bicc1 rescue mRNA. Note enhanced dand5 staining in rescued specimens. C Quantification of dand5 expression after knockdown of bicc1 . The effect was observed in the left and right sLRO cells. D , E Downregulation of nodal1 in bicc1 morphants. D Quantification of results. E Wt specimens show bilateral nodal1 mRNA. Left or right bicc1 SBMO injections reduced nodal1 , which was restored by adding rescue bicc1 mRNA. MO pmol/embryo: bicc1 SBMO (L and S, each 1); bicc1 TBMO, (L and S, each 1); dand5 TPMO (0.5). Asterisks in B and E mark the injected side. Numbers (n) in A , C , and D represent analyzed specimens from more than three independent experiments. Statistical analyses were done with one-sided Pearson’s chi-square test, which was adjusted for multiple comparisons by Bonferroni ( B ) or Bonferroni–Holm ( C , D ). n.s. not significant p > 0.05; * significant, p < 0.05; ** highly significant p < 0.01; ***, very highly significant p < 0.001. p values and listing of individual experiments can be found in the source data file. st., stage. Scale bars in B and E represent 100 µm. st. stage, a anterior, l left, r right, p posterior. Full size image We, therefore, analyzed the expression of the flow target dand5 in post-flow bicc1 morphants. We observed a strong downregulation of dand5 mRNA (Fig. 3B, C ), instead of the expected loss of dand5 repression and blocked mRNA decay. This effect was not restricted to left sLRO cells as right-sided MO injections equally led to dand5 mRNA reduction (Fig. 3C ). In pre-flow stages, dand5 was also downregulated (Supplementary Fig. 3G ). Importantly, dand5 expression was restored in bicc1 morphants by co-injecting bicc1 rescue mRNAs, demonstrating specificity (Fig. 3B, C ). Injecting bicc1 mRNA alone or with MOs boosted dand5 mRNA expression in left or right sLRO cells (Fig. 3B, C ), which hinted towards an enhanced dand5 mRNA stability or expression. Overall, the bicc1 MO phenotype on dand5 mRNA clearly resembled the results obtained when the dand5 3′-UTR was targeted by the m-tpMO (Fig. 2D, E ; Supplementary Fig. 2A ). However, loss of dand5 mRNA by bicc1 LoF was not congruent with observed effects on pitx2 , i.e., no ectopic right-sided induction but the loss of left-sided pitx2 , suggesting that additional factors were affected. To explore this further, we monitored myo1d and confirmed that the positioning and the somitic identity of sLRO cells were unaltered in bicc1 morphants, (Supplementary Fig. 3H ), excluding a general failure in specification or morphogenesis. We then analyzed nodal1 in sLRO cells. Like dand5 , nodal1 expression was substantially reduced in bicc1 morphants at pre- and post-flow stages (Fig. 3D, E ; Supplementary Fig. 3I ). The effect was specific because nodal1 expression was rescued by co-injections of bicc1 mRNAs (Fig. 3D, E ), suggesting that this effect contributed to the observed LR defects, i.e., loss of pitx2 expression. Bicc1 regulation of nodal mRNA has not been reported previously. Taken together, Bicc1 controls the expression of both key effectors of symmetry breakage independent of leftward flow. Bicc1 ensures gdf3 mRNA translation and thereby nodal1 expression Previous reports suggested that nodal1 is regulated by Gdf3 signaling in sLRO cells [31] and that gdf3 is post-transcriptionally regulated [32] . To test whether gdf3 might be regulated by Bicc1, a luciferase reporter containing the gdf3 3′-UTR (361 bp S alloallele) was analyzed in the AC assay. AC cells are devoid of endogenous gdf3 expression. Translation of gdf3 reporter mRNA was significantly repressed by Bicc1 (Fig. 4A ). Unlike dand5 and nodal1 , gdf3 mRNA in sLRO cells was not altered in bicc1 SBMOs injected specimens (Fig. 4B, C ). nodal1 mRNA was diminished in gdf3 morphants leading to impaired pitx2 asymmetry (Supplementary Fig. 4 ), suggesting that Bicc1 could act on gdf3 translation in vivo. If loss of nodal1 mRNA in bicc1 morphants was owing to impaired Gdf3 signaling, nodal1 expression should be restored by gdf3 GoF. Co-injecting bicc1 SBMOs and gdf3 mRNA in the left sLRO lineage indeed rescued nodal1 expression as well as pitx2 asymmetry (Fig. 4 D, E and F, G respectively), demonstrating that Bicc1 enabled Gdf3-dependent nodal1 expression. Thus, in pre-flow stages, Bicc1 seems to be required for securing the interplay of secreted key factors (Nodal1/Gdf3/Dand5) until positional information is provided by leftward flow which represses dand5 . Fig. 4: Bicc1 indirectly regulates nodal1 expression via Gdf3 signaling. A Animal cap assay using a luciferase reporter mRNA which contained gdf3 3′-UTR sequences. Translation of gdf3 reporter was efficiently blocked by co-injecting bicc1 mRNA. N represents the number of independent experiments. A pool of 10 animal caps was analyzed per experiment and treatment. The result from reporter mRNA alone served as a reference and was set to 100% RLU. Relative values of single experiments are depicted as blue dots. Data of three experiments are presented as mean value (bar) ±standard deviation (error bar, SD). Statistical analyses were done with a one-sided Student’s t test for two independent means using the values of three individual experiments. B gdf3 mRNA was not affected by bicc1 LoF. C Quantification of gdf3 expression in bicc1 morphants at the LRO margin. D gdf3 GoF rescues nodal1 expression in bicc1 morphants. Representative nodal1 staining in left sLRO cells is shown for control (co), bicc1 morphant, and rescued specimens. E Quantification of the bicc1 MO rescue of nodal1 expression by gdf3 . F , G Left-asymmetric pitx2 expression (arrowhead) is restored in bicc1 morphants by co-injecting gdf3 mRNA. MO pmol/embryo: bicc1 SBMO (L and S, each 1). Asterisks in B and D mark injected side. Numbers (n) in C , E , and G represent analyzed specimens from more than independent experiments. Statistical analyses were done with one-sided Pearson’s chi-square test, which was adjusted for multiple comparisons by Bonferroni–Holm ( C , E ) or Bonferroni ( G ). n.s. not significant, p > 0.05; ** highly significant p < 0.01; ***, very highly significant p < 0.001. p -values, mean values, SD and listing of individual experiments can be found in the source data file. Scale bars in B and D represent 100 µm and in F 1 mm. RLU relative luciferase units, st. stage, a anterior, l left, r right, p posterior, d dorsal, v ventral. Full size image Bicc1 acts in a context-dependent manner with sub-regions of the Bicc1RE To provide further evidence that Bicc1 regulation of dand5 is relayed through the Bicc1RE, we tested for functional cooperation of bicc1 SBMOs with tpMOs. Consequently, we used single L- or S-specific bicc1 SBMOs which, separately, did not impact on pitx2 , dand5, and nodal1 expression, in combination with suboptimal dosages of tpMOs (Fig. 5A–D ; Supplementary Fig. 3 B, 4A–C ). Right-sided injection of low dose m-tpMO (S or L) together with a single bicc1 SBMO (S or L) resulted in ectopic right-sided LPM induction of pitx2 (Fig. 5A ; Supplementary Fig. 5A ), mimicking treatments with high dose m-tpMO (Fig. 2A, B ). Accordingly, double morphants showed reduced dand5 expression on the injected side (Fig. 5B, C ). These results suggested that in early neurulae dand5 mRNA stability depends on (a) Bicc1 and (b) the accessibility of the medial sub-region of the Bicc1RE. Fig. 5: Bicc1 regulates dand5 mRNA through distinct regions of the Bicc1RE. A Quantification of right-sided pitx2 induction by co-injecting a low, ineffective m-tpMO dosage with single allele-specific bicc1 SBMO. Controls (co), m-tpMO (S or L, low), or allele (S or L) specific bicc1 SBMO alone showed wt pitx2 asymmetry. B Co-injecting m-tpMO (low) with bicc1 TPMO (L or S) impacted dand5 mRNA stability. Treatment with low concentrations of m-tpMO, single allele-specific bicc1 TPMO, and uninjected co showed wt dand5 expression at post-flow stages. C Quantification of dand5 expression. D Quantification of pitx2 asymmetry. Only in combination both suboptimal dosages of d-tpMO (low) or single allele-specific bicc1 SBMO (S or L) prevented left pitx2 expression. Wt expression was found in controls (co) and in embryos that were left-sided injected with one MO alone. MO pmol/embryo: bicc1 SBMO (L or S, 1); m-tpMO low (L or S, 0.4); d-tpMO low (L or S, 0.5). Asterisks in B mark injected side. Numbers (n) in A , C , and D represent analyzed specimens from more than independent experiments. Statistical analyses were done with one-sided Pearson’s chi-square test, which was adjusted for multiple comparisons by Bonferroni ( A , D ) or Bonferroni–Holm ( C ). n.s., not significant p > 0.05; ***, very highly significant p < 0.001. p values and listing of individual experiments can be found in the source data file. Scale bar in B represents 100 µm. st. stage, a anterior, l left, r right, p posterior. Full size image Next, we performed alike experiments with d-tpMOs, to prove the involvement of Bicc1 in post-flow dand5 regulation. Indeed, left-sided injections of low doses of d-tpMO together with allele-specific bicc1 SBMO prevented pitx2 induction in the left LPM (Fig. 5D ; Supplementary Fig. 5B ). Importantly, nodal1 expression in sLRO cells was normal (Supplementary Fig. 5C ), unlike in bicc1 morphants (Fig. 3D, E ). We, therefore, concluded that flow-induced dand5 translational repression required Bicc1 activity, which merged on the distal sub-region of the Bicc1RE. Taken together, the cooperation experiments of bicc1 SBMOs and tpMOs underscore a dual role of Bicc1 on flow independent dand5 mRNA stability or its flow-induced translational repression. Intriguingly, both Bicc1 functions converge on a small 3′-UTR sequence, the Bicc1RE. Bicc1 and Dicer interact in post-transcriptional dand5 regulation Several reports have shown Bicc1 regulation of miRs, small RNAs that bind specific 3′-UTRs and thereby tag the mRNA for translational repression and decay. The RNase III enzyme Dicer processes precursor miRs in the cytoplasm and, together with Ago2, assembles the RNA-induced silencing complex RISC [33] . In the kidney, Bicc1 acted downstream of Dicer1 to transfer target mRNAs unto Ago2, which cleaves or blocks their translation in a miR-dependent manner [22] . To begin exploring the possible role of miRs in dand5 regulation, we analyzed the expression of dicer1 . dicer1 mRNA was expressed in somites and notochord at flow-stage (st. 18; Fig. 6A ). dicer1 mRNA was found specifically in sLRO cells, excluding the cLRO cells in-between and the lateral endodermal cells flanking the LRO (Fig. 6A, A ’). Two MOs that targeted translation (TBMO1 [34] ; TBMO2) through conserved sequences of both S- and L-alleles were used to knockdown dicer . Targeting the left side of the LRO (C2-lineage) inhibited pitx2 expression in the left LPM (Fig. 6B ). Wildtype phenotypes upon right-sided MO injections argue against MO toxicity and off-target effects (Fig. 6B ). A parallel knockdown of dand5 on the left rescued wt pitx2 expression (Fig. 6B ; S6A), further supporting MO-specificity. In addition, western blot analysis confirmed the efficacy of the designed dicer1 TPMO2 (Supplementary Fig. 6B ). In mouse embryos, Dicer was also required for Nodal cascade asymmetry. Induced conditional deletion of Dicer from the mouse LRO prevented the expression of Nodal mRNA in the left LPM (Fig. 6C ). Fig. 6: Dicer interacts with Bicc1 in dand5 repression. A Expression of dicer1 in sensory (s) LRO cells ( N = 3; n = 30) of the frog (GRP; gastrocoel roof plate). Whole-mount in situ hybridizations of stage 18 dorsal explant with a dicer1 -specific antisense RNA probe. (A’) The transverse histological section (indicated in A ) reveals mRNA expression in sLRO cells, somites (som), and deep cells of the notochord (no), but absence of signals from central (c) flow-generating LRO and lateral endodermal cells (end). B Quantification of MO-mediated inhibition of dicer . Note knockdown in left, but not right sLRO cells prevented pitx2 asymmetry in the left LPM, which was rescued by co-injecting dand5 MO. C mRNA expression of nodal in control ( Dicer flox/+ ) and dicer conditional knockout ( Dicer flox/flox Noto CreERT2/+ ) mouse embryos at E8.0. Note that Nodal asymmetry in the left LPM (arrowhead) was lost in mutants. D Absence of flow-induced dand5 mRNA decay at the left LRO margin in post-flow dicer1 morphants (st. 20). Representative dorsal explants of wt (left) and dicer1 morphant (right) specimens hybridized with a dand5 antisense RNA probe. E Quantification of dand5 results. F Flow-induced Dand5 mRNA downregulation in left crown cells of the murine node was lost in Dicer conditional knockout ( Dicer flox/flox Noto CreERT2/+ ) mouse embryos at E7.5. G Lack of dand5 repression in 10 somite stage (ss) MZdicer mutant zebrafish embryos. H Absence of dand5 mRNA by RNAseq reads in 24hpf wt zebrafish embryos, but maintenance in MZ dicer mutants. I bicc1 and dicer1 interact in LR asymmetry. Wt pitx2 expression upon isolated left-sided injections of allele-specific bicc1 SBMOs and moderate effects upon dicer1 TBMO1 injection. Asymmetric pitx2 was significantly inhibited by co-injecting dicer1 and bicc1 MOs. MO pmol/embryo: dicer1 TBMO1 (1.5); dicer1 TBMO2 (1); bicc1 TBMO (L or S, each 1); bicc1 SBMO (L or S, each 1). Asterisks in D mark injected side. Numbers (n) in B , E , and I represent analyzed specimens from three independent experiments. Statistical analyses were done with one-sided Pearson’s chi-square test, which was adjusted for multiple comparisons by Bonferroni ( B , I ) or Bonferroni–Holm ( E ). n.s. not significant p > 0.05; * significant, p < 0.05; ***, very highly significant p < 0.001. p values and listing of individual experiments can be found in the source data file. Scale bars in A , A ’, C , F , and D represent 100 µm. st. stage, a anterior, d dorsal, l left, r right, v ventral, p posterior. Full size image Analyzing earlier stages of laterality determination, left-sided downregulation of Dand5 mRNA levels at post-flow stages was compromised in mouse Dicer mutants and Xenopus dicer1 morphants (Fig. 6D, E, F ). This finding was conserved in zebrafish. In wt 10 somite stage (ss) embryos, dand5 was repressed on the left side of Kupffer’s vesicle (KV), whereas no repression was observed in maternal zygotic dicer mutants (MZ dicer ; Fig. 6G ). At the wt KV dand5 mRNA fades away at 14 ss and is absent at 18 ss (Supplementary Fig. 6C ; source data file). Although MZ dicer mutants showed some developmental delay, dand5 expression was retained as late as 24hpf, which was monitored by ISH (Figure S6C ) and RNAseq (Fig. 6H ; Supplementary Fig. 6D, E ). Loss of dand5 repression upon dicer LoF could be caused by the absence of flow or represent a specific function on dand5 regulation. Previous reports have shown that miRs control motile ciliogenesis [35] , [36] . In agreement with this, ciliation of multiciliated cells in the Xenopus epidermis was impaired in dicer1 morphants (Supplementary Fig. 6H ). When dicer1 MOs were targeted to flow-generating LRO cells (C1-lineage), ciliation was unaltered in morphants (Supplementary Fig. 6F, F’, G ), demonstrating that dicer acted downstream of flow and upstream of dand5 repression, like bicc1 . Next, we investigated whether dicer1 and bicc1 acted in the same pathway in flow-sensing cells. When injecting bicc1 SBMOs (targeting S- or L-alleles) separately, wt pitx2 induction in the left LPM was observed (Fig. 6I ; Supplementary Fig. 3B ). Co-injection of either bicc1 .S- or L-SBMO and dicer1 MO blocked pitx2 expression in ~70% of cases (Fig. 6I ), demonstrating that bicc1 and dicer1 synergize to mediate dand5 repression. Finally, we wondered whether pkd2 , one of two published active components in the flow sensor [37] , [38] , acted in the same pathway. Our recent demonstration of an earlier (likely maternal) Pkd2 function in the specification and morphogenesis of the LRO prevented us from investigating this question in the context of LR axis formation in the embryo itself [28] . In zebrafish, however, zygotic pkd2 mutants and morphants display randomization of nodal ( southpaw ), lefty and pitx2 , but are reported to have normal KV ciliation and morphology [39] , [40] , suggesting a role for Pkd2 in flow sensing. In agreement with this, dand5 mRNA repression was not observed in pkd2 mutant and morphant zebrafish embryos (Fig. 7A, B ), likely being causative for misregulation of the Nodal cascade in these backgrounds [39] . To test a potential interplay between pkd2 and bicc1 in the process of dand5 repression, we returned to the Xenopus AC assay (Fig. 1A ). In order to record additive effects of pkd2 , we attenuated the Bicc1-mediated repression of the dand5 reporter by lowering the concentration of co-injected bicc1 mRNA, such that reporter activity was only repressed to ~40% of wt-level (Fig. 7C ). Upon co-injection of full-length pkd2 mRNA, reporter activity was further repressed to under 20% (Fig. 7C ). pkd2 mRNA alone, however, increased the reporter mRNA’s expressivity fourfold. Because pkd2 is maternally expressed in animal tissue, like dand5 , we tested this interaction further by co-injecting pkd2 MO, the specificity of which we showed previously [17] , [41] . Loss of pkd2 partially rescued bicc1 -mediated repression of the dand5 reporter (Fig. 7C ), which again is contrasted in a bicc1 free set up, where pkd2 is required for efficient translation. Therefore, these experiments underscore a scenario in which an upstream ion-channel Pkd2 is able to modulate Bicc1 function during post-transcriptional regulation of dand5 . Fig. 7: Pkd2 function modifies Bicc1-mediated translational repression of dand5 . A Absence of dand5 repression in maternal zygotic (MZ) pkd2 mutant zebrafish at 10 somite stage (ss). B Quantification of dand5 asymmetry in controls (co) and pkd2 morphant (1–4 ng) zebrafish. Asymmetry was determined by picture analysis using ImageJ. Number (n) represents the number of analyzed specimens. Statistical analyses were done with one-sided Pearson’s chi-square test. 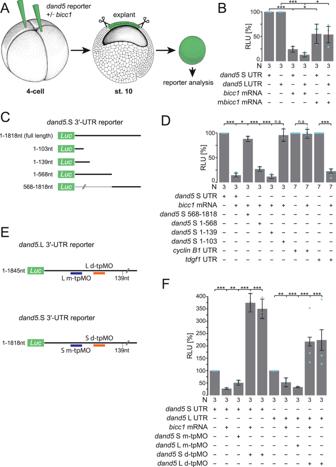C Animal cap luciferase reporter assay of full-length dand5.S 3′-UTR (cf. Fig. 1: Bicc1 repressesdand5mRNA translation via its proximal 3′-UTR. ASchematic depiction ofdand5reporter assay.dand53′-UTR sequences fused to luciferase coding were injected either with or withoutbicc1mRNA into the animal region of four-cell embryos. At st. 10, the animal cap region was excised and assayed for luciferase activity. Adapted from refs.65and66.BAnimal cap reporter assay following injections ofdand5S- or L 3′-UTRs alone or together withXenopus(bicc1) or mouseBicc1(mbicc1) effector mRNAs. Note that both alloalleles were equally repressed. Note also thatmbicc1was efficient as a repressor as well.CLuciferase reporter constructs harboring different regions of thedand5(S-allele) 3′-UTR.DRepression of translation is mediated through a proximal 139 nucleotides (nt) sequence element in thedand53′-UTR.ESchematic depiction of medial and distal target protector MOs (m-tpMOs or d-tpMOs) binding to the minimal Bicc1 responsive element (Bicc1RE) in thedand53′-UTR (L or S).Fm- and d-tpMOs (0.4 or 0.5 pmol/embryo, respectively) interact differently with the luciferase reporter expression. m-tpMO blocked and d-tpMO boosted luciferase activity. Co-injection of d-tpMOs prevented Bicc1-dependent repression of the full-lengthdand5reporters (L and S) and further enhanced their expressivity. N inB,D, andFrepresents the number of independent experiments. A pool of 10 animal caps was analyzed per experiment and treatment. Results from reporter mRNAs alone served as reference and were set to 100% RLU. Relative values of single experiments are depicted as blue dots. Data of at least three experiments are presented as mean value (bar) ±standard deviation (error bar, SD). Statistical analyses were done with a one-sided Student’sttest for two independent means (Bonferroni corrected) using the values of at least three individual experiments.pvalues, values for individual experiments, the mean values, and standard deviations are found in the source data file. n.s. not significantp> 0.05; * significant,p< 0.05; ** highly significantp< 0.01; ***, very highly significantp< 0.001; RLU relative luciferase units;Lucluciferase. Figure 1A ). The reporter construct was injected as mRNA either alone or in combination with high or low dose bicc1 mRNA, pkd2 mRNA or pkd2 TBMO. Gradual repression upon co-injection of high or low concentrations of bicc1 mRNA was observed. Administering only pkd2 mRNA or pkd2 TBMO (1 pmol) efficiently blocked or boosted luciferase expression, respectively. The data further indicate that in AC cells endogenous dand5 mRNA is post-transcriptionally regulated in a Pkd2-dependent manner. In the presence of a lower amount of bicc1 mRNA high-level, strong repression was achieved when pkd2 mRNA was co-injected, or further diminished upon knockdown of pkd2 using TBMO. N represents the number of independent experiments. A pool of 10 animal caps was analyzed per experiment and treatment. The results from reporter mRNA alone served as reference and were set to 100% RLU. Relative values of single experiments are depicted as blue dots. Data of three experiments are presented as mean value (bar) ±standard deviation (error bar, SD). Statistical analyses were done with a one-sided Student’s t test for two independent means (Bonferroni corrected) using the values of three individual experiments. p values, values for individual experiments, mean values, and standard deviations are found in the source data file. n.s. not significant, p < 0.05; ** highly significant p < 0.01; ***, very highly significant p < 0.001, RLU relative luciferase units, Luc luciferase . Full size image In summary, data presented here demonstrate that the proximal dand5 3′-UTR contains regulatory sequences, which allow the RNA-binding protein Bicc1 and the miR-processing enzyme Dicer to execute flow-dependent dand5 repression. Thereby this Bicc1RE likely reflects the downstream target of calcium released by Pkd2 in sensing of leftward flow at the left LRO margin. We have identified a minimal 139 nt sequence in the dand5 3′-UTR, which was sufficient to mediate Bicc1-dependent post-transcriptional regulation. This Bicc1RE contains two sub-regions, medial and distal, which represent two distinct regulatory entities in a pre- and post-flow setting. In pre-flow stages, free access to the medial sub-region and a sufficient amount of Bicc1 protein was required to maintain dand5 mRNA expression. In this  context, Bicc1 might protect dand5 against premature mRNA decay and ensures Dand5 protein synthesis. However, observed LR defects in bicc1 morphants were to a great extent caused by loss of nodal1 expression, which so far has not been reported in other organisms. We identified an additional potential Bicc1 target, the Tgfβ ligand gdf3 . This was evidenced by the efficient repression of the gdf3 3′-UTR reporter mRNA by Bicc1 (Fig. 4A ). However, gdf3 mRNA expression, unlike dand5 and nodal1 , was not impaired by bicc1 LoF indicating that in this case, Bicc1 acted on translation only. 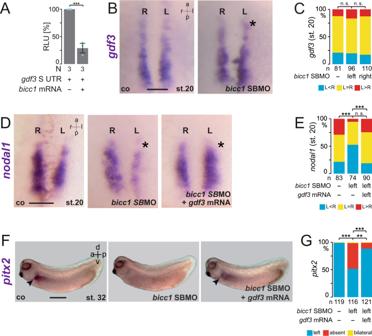Fig. 4: Bicc1 indirectly regulates nodal1 expression via Gdf3 signaling. AAnimal cap assay using aluciferasereporter mRNA which containedgdf33′-UTR sequences. Translation ofgdf3reporter was efficiently blocked by co-injectingbicc1mRNA. N represents the number of independent experiments. A pool of 10 animal caps was analyzed per experiment and treatment. The result from reporter mRNA alone served as a reference and was set to 100% RLU. Relative values of single experiments are depicted as blue dots. Data of three experiments are presented as mean value (bar) ±standard deviation (error bar, SD). Statistical analyses were done with a one-sided Student’sttest for two independent means using the values of three individual experiments.Bgdf3mRNA was not affected bybicc1LoF.CQuantification ofgdf3expression inbicc1morphants at the LRO margin.Dgdf3GoF rescuesnodal1expression inbicc1morphants. Representativenodal1staining in left sLRO cells is shown for control (co),bicc1morphant, and rescued specimens.EQuantification of thebicc1MO rescue ofnodal1expression bygdf3.F,GLeft-asymmetricpitx2expression (arrowhead) is restored inbicc1morphants by co-injectinggdf3mRNA. MO pmol/embryo:bicc1SBMO (L and S, each 1). Asterisks inBandDmark injected side. Numbers (n) inC,E, andGrepresent analyzed specimens from more than independent experiments. Statistical analyses were done with one-sided Pearson’s chi-square test, which was adjusted for multiple comparisons by Bonferroni–Holm (C,E) or Bonferroni (G). n.s. not significant,p> 0.05; ** highly significantp< 0.01; ***, very highly significantp< 0.001.p-values, mean values, SD and listing of individual experiments can be found in the source data file. Scale bars inBandDrepresent 100 µm and inF1 mm. RLU relative luciferase units, st. stage, a anterior, l left, r right, p posterior, d dorsal, v ventral. Gdf3 is required for efficient Nodal diffusion and therefore LR patterning [16] , [31] , [42] , [43] . In Xenopus sLRO cells an additional gdf3 function was reported, suggesting that Gdf3 signaling is upstream of nodal1 transcription [32] , which we validated in this study (Supplementary Fig. S4A, B ). This finding was underscored by our observation that gdf3 overexpression restored nodal1 expression in bicc1 morphants. Currently, there is no evidence of such a mechanism in other vertebrates and it likely reflects a frog-specific feature. We propose a pre-flow situation in which Bicc1 safeguards the expression of dand5 and gdf3 in a post-transcriptional manner. Thus, it indirectly influences nodal1 transcription via Gdf3 signal transduction (Fig. 8 ). In the embryonic kidney of Xenopus , a comparable protective Bicc1 function was shown for pkd2 [17] . Such a scenario should be relevant to ensure an at least equimolar equilibrium of the inhibitor Dand5 and its targets in sLRO cells. In addition, Bicc1 control of gdf3 limits or prevents ectopic Nodal signaling and premature Nodal/Gdf3 diffusion until flow sensing. Fig. 8: Two modes of Bicc1-dependent post-transcriptional regulation of gdf3 and dand5 in flow sensor cells at the Xenopus left-right organizer. In the early neurula pre-flow stages, Bicc1 has two functions. Bicc1 assures gdf3 mRNA translation and thereby indirectly ensures nodal1 transcription by Gdf3 signaling. Simultaneously Bicc1 mediates dand5 mRNA stability via the medial (m) sub-region of the Bicc1RE. Thus, Dand5 protein levels are sustained on both sides, keeping Nodal in tight repression. Leftward flow activates the Pkd2 channel in left flow sensor cells, resulting in an asymmetric calcium signal. In post-flow stages, a calcium-dependent mechanism activates/modifies Bicc1 to become a repressor of dand5 translation, which is relayed by the distal (d) sub-region of the Bicc1RE. Subsequently, dand5 mRNA gets degraded in a Dicer1 (miR) dependent manner. Attenuated Dand5 expression lifts repression of Nodal and defines leftness by induction of the LPM Nodal signaling cascade. For details, see text. Full size image Early Bicc1 functions impeded the analysis of flow-dependent dand5 mRNA regulation, but we were able to show several lines of evidence that Bicc1 serves as the critical mediator of flow sensing and primarily blocks dand5 translation. (1) Rescue of pitx2 asymmetry in bicc1 morphants by dand5 knockdown demonstrated that even when dand5 and nodal1 were strongly reduced, dand5 was not repressed in absence of Bicc1. (2) Using our d-tpMOs, we separated dand5 mRNA decay from translation inhibition: left-sided, flow-dependent dand5 mRNA reduction was still observed in d-tpMO morphants (Fig. 2G, H ), whereas left nodal cascade induction was inhibited (Fig. 2A, C ). (3) Bicc1 dosage and availability of distal sequences of the Bicc1RE cooperated in flow-dependent dand5 repression and left pitx2 LPM induction, without any effects on dand5 mRNA stability (Fig. 5D ; Supplementary Fig. 5D ). (4) The accompanying manuscript by Minegishi et al. [44] demonstrates Bicc1 binding to the mouse Dand5 3′-UTR and identified specific binding motifs. Intriguingly, we found alike sequences in the Bicc1RE, which apparently were located within dS-tpMO or next to dL-tpMO target sequences that specifically impair translational repression in Xenopus (Figure S1B ). In addition, deleting the distal 36 nucleotides of the Bicc1RE, which contains the site, renders the dand5 reporter mRNA insensitive to Bicc1 (Fig. 1D ). Based on the conserved nature of dand5 as the flow target, the finding in mouse should also apply to Xenopus . Potential sites were also found in the gdf3 3′-UTR, underscoring their relevance. (5) Both Bicc1 and Dicer are well known for post-transcriptional regulation and they functionally interacted in flow-induced dand5 repression (Fig. 6I ). (6) The flow sensor pkd2 was able to modulate Bicc1 properties on dand5 translational inhibition, suggesting that calcium could serve as the switch from a safeguarding pre-flow to a modified inhibitory post-flow Bicc1 function. Our work, together with complementing analyses in the mouse (cf. [44] ), constitutes a conceptual advance in our understanding of symmetry breaking, namely the flow-dependent activation of the RNA-binding protein Bicc1 to repress dand5 translation on the left LRO margin in a Dicer-dependent manner. Based on our analyses, we suggest a model schematically depicted in Fig. 8 . In the pre-flow scenario, Bicc1 protects dand5 mRNA in a bilateral symmetric manner, which is relayed by the medial sub-region of the Bicc1RE. Thereby, Dand5 synthesis and Nodal inhibition are secured. During flow, left-sided Pkd2 channel activation results in a cytoplasmic Ca 2+ signal, which has been described in mouse and zebrafish [10] , [11] , [38] , [45] , [46] . It represents the intracellular second messenger of the initially extracellular flow signal. In zebrafish, transient activation of CaMK-II downstream of asymmetric Ca 2+ is required in the LRO for asymmetric Nodal cascade induction and correct development of organ situs [47] . We hypothesize that Bicc1 gets functionally modified (Bicc1*) by Pkd2 and potentially Ca 2+ , which alters Bicc1 properties from initial dand5 mRNA stabilization to translation inhibition, followed by mRNA decay (Fig. 8 ). How this molecular switch is achieved remains unclear. In Drosophila, Bicc1 phosphorylation has been reported and therefore Ca 2+ -dependent phosphorylation might lead to functional changes [48] . Then again, under certain conditions, Bicc1 is thought to form polymeric complexes. Recently it was speculated that monomeric or polymeric Bicc1 aggregates may act differentially on post-transcriptional regulation. It was proposed that in left sLRO cells Bicc1 polymerization might be induced in a pkd2 /Ca 2+ -dependent manner that blocks dand5 translation, whereas on the right side only low molecular Bicc1 complexes are present, allowing Dand5 synthesis [49] . So far, we do not have any evidence of how Bicc1 is modified by the leftward flow. However, our analysis demonstrated that the functional switch is accompanied by a differential requirement of relevant sub-regions in the 3′-UTR of dand5 . This finding may be very useful in the future to map crucial Bicc1 domains and sequences for dand5 inhibition. In evolutionary terms, the pkd2 / bicc1 / dicer module is functionally conserved from zebrafish to mammals. In mouse and Xenopus , a proximal element of the dand5 3′-UTR is required and sufficient for flow-mediated mRNA decay and translational inhibition, respectively, which is dependent on Bicc1 and Dicer (cf. [44] ). Whether or not miRs are involved in Dicer1-mediated dand5 repression remains open. The analysis of the proximal regions of various vertebrate dand5 3′-UTR sequences, which show the highest degree of conservation, using different miR-target prediction tools, detects only a few potential miR-binding sites, with low probabilities in all cases. However, miR-133 may be relevant, because members of this family are specific for muscle development and expressed in somites and sLRO cells have somitic fate [8] , [50] , [51] , [52] . A conserved target site was detected in the Bicc1RE of X. laevis S- and L-alleles and the human proximal dand5 3′-UTR (Figure S1B ; Supplementary Fig. 7A ). It remains to be seen whether one of the four family members in Xenopus is involved in Bicc1-mediated dand5 mRNA stability and post-flow repression. Interestingly, Bicc1 regulates its own expression in a post-transcriptional manner [53] . A highly conserved miR-133-binding site in 3′-UTRs of vertebrate bicc1 genes (Supplementary Fig. 7A, B, C ) may suggest that a Bicc1/miR-133 module has been adapted to the regulation of dand5 in somitic/sLRO cells. Alternatively, Dicer may act miR-independently through one of its described non-canonical mechanisms [54] . In conclusion, our work identified Bicc1 and Dicer as two factors downstream of leftward flow sensing. The exact nature of Bicc1’s modifications and interactions with the dand5 Bicc1RE in a pre-flow and post-flow setting remains to be solved. Image processing Imagej (1.48i), Acrobat Illustrator (cs6), and Acrobat Photoshop (cs6) were used for image processing. Plasmid construction The m bicc1 -CS2+ construct was a gift from Oliver Wessely (Cleveland, OH, United States). 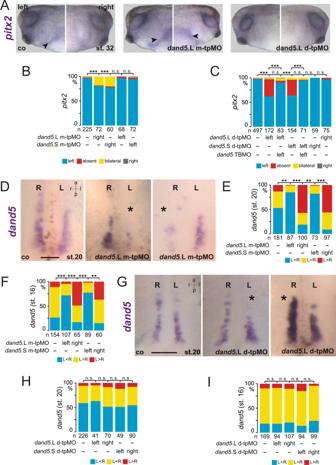For in vitro synthesis of mRNA using the Ambion sp6 message kit, the plasmids were linearized with NotI. Firefly luciferase reporter mRNAs that contained the gdf3 mRNA 3′-UTR (GenBank: BC073508.1) or the 3′-UTR of the dand5 .L mRNA or the dand5 .S mRNA the Ambion T7 message kit were used and the plasmids were linearized with BamH1. Fig. 2: Bicc1 responsive element (Bicc1RE) of thedand53′-UTR is required for LR asymmetry. AUninjected control (co), m-tpMO, or d-tpMO-injected embryos showed left, bilateral, or absentpitx2expression, respectively. Lateral views (left and right) of embryos are presented. Arrowheads markpitx2-positive lateral plate mesoderm.BQuantification ofpitx2results of m-tpMO-treated specimens.CQuantification ofpitx2asymmetry by d-tpMO injections. Note administration ofdand5TPMO together with d-tpMOs restored wtpitx2expression.DDiminisheddand5mRNA expression by left-sided and right-sided m-tpMO injections compared with control.EQuantification ofdand5expression at post-flow stages (st.20) following m-tpMO treatment.FQuantification ofdand5expression in pre-flow specimens injected with m-tpMO.GWildtypedand5repression in control (co) and left- or right-sided d-tpMO injected specimens.HQuantification ofdand5asymmetry. Note flow-induceddand5mRNA decay was observed in controls and following d-tpMO application.IQuantification ofdand5staining of pre-flow specimens (st.16) following d-tpMO injections. MO pmol/embryo: m-tpMO (L or S, 0.8); d-tpMO (L or S, 1). Asterisks inDandGmark injected side. Scale bars inDandGrepresent 100 µm. Numbers (n) inB,C,E,F,H, andIrepresent analyzed specimens from more than three independent experiments. Statistical analyses were done with one-sided Pearson’s chi-square test, which was adjusted for multiple comparisons by Bonferroni (B,C) or Bonferroni–Holm (E,F,H,I).pvalues and listing of individual experiments can be found in the source data file. n.s. not significantp> 0.05; **highly significantp< 0.01; ***very highly significantp< 0.001; st. stage; a anterior; l left; r right; p posterior. Supplemental Table 2 lists all primers with sequences used in the context of this work. RT-PCR RT-PCR was conducted using either the L or S isoform-specific primer for intron 2 or intron 1, respectively, and an isoform-specific reverse primer in exon 5 with 38 cycles. The listing of individual primers used in this work can be found in Supplemental Table 2 . Morpholinos Supplemental Table 1 lists all MOs used with references to previous validations or proof of specificity in the context of this work. Xenopus frogs and embryos Animals were handled in accordance with German regulations (Tierschutzgesetz) and approved by the Regional Council Stuttgart (A379/12 Zo, ‘Molekulare Embryologie’, V340/17 ZO and V349/18 ZO, ‘ Xenopus Embryonen in der Forschung’). Xenopus embryos obtained by in vitro fertilization were maintained in 0.1× modified Barth medium [55] and staged according to ref. [56] . During injections, embryos were kept in 1× modified Barth medium with 2% Ficoll. To specifically target the sensory cells of the GRP for all experiments except for the luciferase assay, we injected them into the dorsal marginal side (left or right; C2-lineage). For luciferase assays, embryos were injected twice into the animal blastomeres at the four-cell stage with a luciferase dand5 3′-UTR construct, alone or together with a bicc1 construct. Animal cap tissue was dissected at stage 10 (cf. Figure 1A for a schematic depiction of the procedure). Following injections, all embryos were transferred to 0.1 modified Barth medium. Zebrafish Established husbandry protocols were adhered to, and experimental protocols were conducted, in accordance with the Princeton University Institutional Animal Care and Use Committee (IACUC) guidelines. Zebrafish strains utilized include pkd2/cup tc321 [39] and dicer1 hu715 [57] . The pkd2 AUG MO is described in ref. [39] . Embryos were staged according to ref. [58] . Embryos were raised at 28 °C and processed for injections. For all knockdowns, a morpholino mixture of ~1.8 nl was injected into the yolk of one-cell stage embryos. All morpholino mixtures contained Danieau’s Buffer and 0.5 mg/ml phenol red. Embryos were fixed at the 10 ss stage in 4% paraformaldehyde (PFA) overnight at 4 °C. These embryos were washed with PBST (1× PBS containing 0.1% Tween 20), dechorionated, transitioned to 100% methanol, and stored at −20 °C for at least 1 day. The transition to methanol was done by performing 5-minute washes in 75% 1× PBST:25% methanol, 50% 1× PBST:50% methanol, 25% 1× PBST:75% methanol, and 100% methanol. The embryos were then transitioned into 1× PBST by performing 5 min washes in 25% 1× PBST:75% methanol, 50% 1× PBST:50% methanol, and 75% 1× PBST:25% methanol. Embryos were then washed four times in 1× PBST with 5 min per wash. Somite stage embryos were incubated for 1 min in 1× PBST containing 0.01 mg/ml Proteinase K (Sigma Aldrich, P2308) followed by a 20 min incubation in 1× PBST containing 4% PFA. These embryos were then washed five more times in 1× PBST with 5 min per wash. Blastula and gastrula stage embryos did not undergo this Proteinase K treatment, extra fixation with 4% PFA, or the extra five washes with 1× PBST. Embryos were incubated in HYB (50% formamide, 5× SSC, 500 µg/ml torula yeast RNA, 50 µg/ml heparin 0.1% Tween 20, and 9 mM Citric Acid (pH 6.0)) for 2 h at 68 °C. Embryos were then incubated overnight in HYB containing an ISH probe at 68 °C. The next day, embryos were washed at 68 °C in HYB, 75% HYB: 25% 1× SSC, 50% HYB: 50% 1× SSC, 25% HYB: 75% 1× SSC, and 1× SSC for 10 min each wash. Embryos were then washed twice in 0.1× SSC for 30 min each wash. The remaining washes were performed at room temperature. Embryos were washed in 75% 0.1× SSC: 25% 1× PBST, 50% 0.1× SSC: 50% 1× PBST, 25% 0.1× SSC: 75% 1× PBST, and 1× PBST for 5 min each wash. Next, embryos were incubated on a rocker for 2 h in 1× PBST containing 2 mg/ml bovine serum albumin (BSA) and 2% normal sheep serum (NSS). Embryos were then incubated overnight on a rocker in 1× PBST containing 2 mg/ml BSA, 2% NSS, and 1:3500 of Anti-Digoxigenin-AP (Roche, 11093274910). The next day, the embryos were washed quickly in 1× PBST followed by six additional 15 min 1× PBST washes on a rocker. Embryos were then washed three times in NTMT (0.1 M Tris-Cl ph 9.5, 0.1 M NaCl, 0.05 M MgCl 2 , 0.1% Tween 20) and stained with 5 µl of NBT (Roche, 11383213001) and 3.75 µl BCIP (Roche, 11383221001) per 1 ml of NTMT. Staining was stopped by washing the embryos three times with NTMT, a 5 min wash with 1× PBST, and a 4 °C overnight incubation in 1× PBST containing 4% PFA. The embryos were then transitioned to methanol using the same four-step PBST:methanol washes listed above. Embryos were stored at −20 °C or cleared in 2:1 Benzyl Benzoate:Benzyl Alcohol prior to imaging. Canada Balsam containing 10% methyl salicylate was used to mount cleared embryos on a slide. RNA ISH staining was visualized using a Leica DMRA2 microscope and images were acquired using a Leica DFC450 C camera. The following probes were used for the ISHs: dand5 . ImageJ RNA ISH image analysis of Zebrafish embryos Pictures taken of the U-shaped dand5 domain were cropped in Adobe Photoshop into equal-sized regions of interest corresponding to the left and right sides of the domain. The center of the domain was used as the midline for generating the left and right domains, and the entire staining area was included in the subsequent quantification analysis. “Subtract Background” in ImageJ 1.48i was used to remove unwanted background signals and images were inverted such that a darker stain, relating to more RNA presence, would yield a higher intensity. A ratio was obtained by dividing the right intensity by the left intensity. In this analysis, a right-biased dand5 domain would have a ratio of 1.1 or higher, a left-biased dand5 domain would have a ratio of 0.9 or lower, and an equal dand5 domain would have a ratio between 0.9 and 1.1. At each stage and condition noted, the indicated number of embryos examined is mentioned as the n value. To minimize any image saturation bias, RNA in situ staining reactions were carefully monitored and stopped when the dand5 domain was first evident. RNAseq Raw reads were mapped to the zebrafish GRCz11 genome using STAR version 2.7.3a [59] with the following non-default parameters: ╌alignEndsType ╌Local ╌outFilterMultimapNmax 1000 ╌seedSearchStartLmax 30 ╌sjdbScore 2–outMultimapperOrder Random. 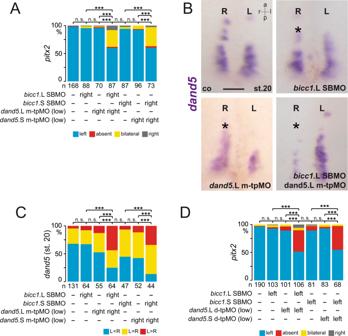Fig. 5: Bicc1 regulatesdand5mRNA through distinct regions of the Bicc1RE. AQuantification of right-sidedpitx2induction by co-injecting a low, ineffective m-tpMO dosage with single allele-specificbicc1SBMO. Controls (co), m-tpMO (S or L, low), or allele (S or L) specificbicc1SBMO alone showed wtpitx2asymmetry.BCo-injecting m-tpMO (low) withbicc1TPMO (L or S) impacteddand5mRNA stability. Treatment with low concentrations of m-tpMO, single allele-specificbicc1TPMO, and uninjected co showed wtdand5expression at post-flow stages.CQuantification ofdand5expression.DQuantification ofpitx2asymmetry. Only in combination both suboptimal dosages of d-tpMO (low) or single allele-specificbicc1SBMO (S or L) prevented leftpitx2expression. Wt expression was found in controls (co) and in embryos that were left-sided injected with one MO alone. MO pmol/embryo:bicc1SBMO (L or S, 1); m-tpMO low (L or S, 0.4); d-tpMO low (L or S, 0.5). Asterisks inBmark injected side. Numbers (n) inA,C, andDrepresent analyzed specimens from more than independent experiments. Statistical analyses were done with one-sided Pearson’s chi-square test, which was adjusted for multiple comparisons by Bonferroni (A,D) or Bonferroni–Holm (C). n.s., not significantp> 0.05; ***, very highly significantp< 0.001.pvalues and listing of individual experiments can be found in the source data file. Scale bar inBrepresents 100 µm. st. stage, a anterior, l left, r right, p posterior. Genomic sequence indices for STAR were built using exon-junction coordinates from Ensembl r92 [60] . Read counts per protein-coding gene were computed by summing the total number of reads overlapping the gene annotation by at least 10 nucleotides. All reads were used and contributed for 1/(number of mapping loci) to the gene counts. Per gene annotation was obtained by concatenating all Ensembl isoforms together. A total number of reads mapping to protein-coding genes and their lengths were used to normalize to RPKM (Reads Per Kilobase per Million mapped reads). For comparison, the average RPKMs of the following house-keeping genes were calculated: actb1 (Actin, beta 1; cytoskeletal), arpc2 (Actin related protein complex; cytoskeletal), eif2a (Eukaryotic translation initiation factor 2 A; translation), ddx39b (DEAD box polypeptide 39B; RNA splicing), pabpn1 (Poly(A) binding protein, nuclear 1; RNA splicing), and rps6 (Ribosomal protein S6; ribosomal protein). LabxDB [61] was employed to manage sequencing samples. Immunofluorescence staining For immunofluorescence staining, embryos were fixed in 4% PFA for 1 h at RT on a rocking platform, followed by 2 washes in 1× PBS − for 15 min each. For staining of LRO explants, embryos were dissected using a scalpel into anterior and posterior halves. Posterior halves (LRO explants) were collected and transferred to a 24-well plate and washed twice for 15 min in PBST. LRO explants and whole embryos were blocked for 2 h at RT in CAS-Block diluted 1:10 in PBST. The blocking reagent was replaced by an antibody solution (anti-acetylated tubulin antibody, diluted 1:700 in CAS-Block; c2181 Sigma) and incubated overnight at 4 °C. In the morning, the antibody solution was removed and explants/embryos were washed twice for 15 min in PBS − . The secondary antibody (diluted 1:1000 in CAS-Block; c2181 Sigma) was added together with Phalloidin (1:200) and incubated for a minimum of 3 h at RT. Before photo documentation, embryos or explants were briefly washed in PBS − and transferred onto a microscope slide. Western blot Embryos were lysed with 10 µl/embryo RIPA buffer (radio immuno precipitation assay buffer) and centrifuged at maximum speed for 15 min at 4 °C and the supernatant was transferred into a new tube. The supernatant was boiled with 1× Laemmli Loading Buffer for 5 min at 95 °C. Probes were transferred to a 4–20% sodium dodecyl sulfate (SDS) gel (BIO RAD Mini-PROTEAN TGX Gels) and gel ran for 1 h at 120 V on a BIO RAD Mini-PROTEAN Tetra System. SDS Gel and nitrile-cellulose membrane were equilibrated in blotting buffer for 30 min and blotted for 1 h at 350 mA. The membrane was dissected and blocked (5% milk powder in Tbs t ) for 1 h at room temperature. Incubation with primary antibodies (monoclonal anti-α-tubin produced in mouse, Sigma Aldrich T9026, 1:3000; monoclonal anti-Dicer1 produced in mouse, BioLegend MMS5130, 1:100) overnight at 4 °C. Membranes were washed in blocking solution (5% milk powder in Tbs t ) and incubated with 2° antibody (Anti-Mouse IgG-peroxidase, Sigma Aldrich A9044, 1:80.000) for 3 h at room temperature. Antibody was removed and membranes were washed with Tbs t and developed using Pierce ECL Western Blotting Substrate (ThermoScientific, #362109) and recorded with an exposure time of 600 µs. Uncropped blots can be found in the source data file. Luciferase assay Luciferase reporter assays were carried out using the Promega Dual-Luciferase® Reporter Assay System. Animal cap tissue, derived from 10 embryos per treatment, was transferred into a 1.5 ml Eppendorf tube, and the 0.1× MBSH buffer was removed, leaving the tissue moistened. The tissue was lysed and homogenized in 100 µl 1× passive lysis buffer by pipetting the suspension up and down, followed by 15 min incubation at RT. The lysate was centrifuged for 2 min at 21,951 × g and the upper phase was transferred into a new tube. The lysate was re-centrifuged and two 25 µl aliquots (technical duplicates) of each sample were transferred into a 96-well plate. 75 µl 1× Luciferase assay substrate was added through the GloMax® Explorer System and luminescence was determined. This step was repeated with 75 µl 1× Stop and Glow reagents. To calculate the relative luciferase units (RLU [%]), the ratio between luciferase and Renilla values was calculated and correlated to the wt control, which was set to 100%. Each sample was measured twice to validate the technical aspect of testing. In order to be valid, the technical replicates should have almost identical values, which was true in all our experiments. Statistics and reproducibility Statistical calculations of marker gene expression patterns and cilia distribution were performed using one-sided Pearson’s chi-square test in statistical R. Adjustments for multiple comparisons were done by Bonferroni ( pitx2 expression) or Bonferroni–Holm ( nodal1 and dand5 expression) corrections. For the statistical calculation of ciliation, a Wilcoxon-Match-Pair test was used (statistical R-3.0.1). Statistical calculations of the luciferase assays were done with a one-sided student’s t test for two independent means in statistical R. Bonferroni corrections were implemented when multiple comparisons were conducted. At least three independent successful biological replicates (embryo batches) were used for each experimental setup. The source data file depicts all individual experiments/data points, mean values with standard deviations, and p values. Mouse strains All mouse experiments were performed in accordance with guidelines of the RIKEN Center for Biosystems Dynamics Research (BDR) and under an institutional license (A2016-01-6). Mice were maintained in the animal facility of the RIKEN Center for BDR. Noto-Cre ERT2 mice were described in ref. [62] , Dicer flox mice in ref. [63] (JAX stock #006001). Expression of the Noto-Cre ERT2 transgene in embryos was induced by oral administration of tamoxifen (Sigma) in corn oil to pregnant mice at a dose of 5 mg both 24 and 12 h before the late headfold stage. WISH analysis in mouse WISH was performed according to standard procedures with digoxigenin-labeled riboprobes specific for Nodal or Dand5 mRNA [64] . 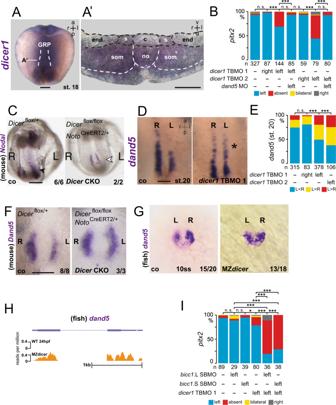Fig. 6: Dicer interacts with Bicc1 indand5repression. AExpression ofdicer1in sensory (s) LRO cells ( N = 3; n = 30) of the frog (GRP; gastrocoel roof plate). Whole-mount in situ hybridizations of stage 18 dorsal explant with adicer1-specific antisense RNA probe. (A’) The transverse histological section (indicated inA) reveals mRNA expression in sLRO cells, somites (som), and deep cells of the notochord (no), but absence of signals from central (c) flow-generating LRO and lateral endodermal cells (end).BQuantification of MO-mediated inhibition ofdicer. Note knockdown in left, but not right sLRO cells preventedpitx2asymmetry in the left LPM, which was rescued by co-injectingdand5MO.CmRNA expression ofnodalin control (Dicerflox/+) anddicerconditional knockout (Dicerflox/floxNotoCreERT2/+) mouse embryos at E8.0. Note thatNodalasymmetry in the left LPM (arrowhead) was lost in mutants.DAbsence of flow-induceddand5mRNA decay at the left LRO margin in post-flowdicer1morphants (st. 20). Representative dorsal explants of wt (left) anddicer1morphant (right) specimens hybridized with adand5antisense RNA probe.EQuantification ofdand5results.FFlow-inducedDand5mRNA downregulation in left crown cells of the murine node was lost inDicerconditional knockout (Dicerflox/floxNotoCreERT2/+) mouse embryos at E7.5.GLack ofdand5repression in 10 somite stage (ss) MZdicer mutant zebrafish embryos.HAbsence ofdand5mRNA by RNAseq reads in 24hpf wt zebrafish embryos, but maintenance in MZdicermutants.Ibicc1anddicer1interact in LR asymmetry. Wtpitx2expression upon isolated left-sided injections of allele-specificbicc1SBMOs and moderate effects upondicer1TBMO1 injection. Asymmetricpitx2was significantly inhibited by co-injectingdicer1andbicc1MOs. MO pmol/embryo:dicer1TBMO1 (1.5);dicer1TBMO2 (1);bicc1TBMO (L or S, each 1);bicc1SBMO (L or S, each 1). Asterisks inDmark injected side. Numbers (n) inB,E, andIrepresent analyzed specimens from three independent experiments. Statistical analyses were done with one-sided Pearson’s chi-square test, which was adjusted for multiple comparisons by Bonferroni (B,I) or Bonferroni–Holm (E). n.s. not significantp> 0.05; * significant,p< 0.05; ***, very highly significantp< 0.001.pvalues and listing of individual experiments can be found in the source data file. Scale bars inA,A’,C,F, andDrepresent 100 µm. st. stage, a anterior, d dorsal, l left, r right, v ventral, p posterior. 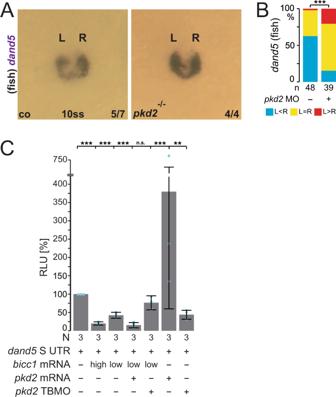Fig. 7: Pkd2 function modifies Bicc1-mediated translational repression ofdand5. AAbsence ofdand5repression in maternal zygotic (MZ)pkd2mutant zebrafish at 10 somite stage (ss).BQuantification ofdand5asymmetry in controls (co) andpkd2morphant (1–4 ng) zebrafish. Asymmetry was determined by picture analysis using ImageJ. Number (n) represents the number of analyzed specimens. Statistical analyses were done with one-sided Pearson’s chi-square test.CAnimal cap luciferase reporter assay of full-lengthdand5.S3′-UTR (cf. Figure1A). The reporter construct was injected as mRNA either alone or in combination with high or low dosebicc1mRNA,pkd2mRNA orpkd2TBMO. Gradual repression upon co-injection of high or low concentrations ofbicc1mRNA was observed. Administering onlypkd2mRNA orpkd2TBMO (1 pmol) efficiently blocked or boosted luciferase expression, respectively. The data further indicate that in AC cells endogenousdand5mRNA is post-transcriptionally regulated in a Pkd2-dependent manner. In the presence of a lower amount ofbicc1mRNA high-level, strong repression was achieved whenpkd2mRNA was co-injected, or further diminished upon knockdown ofpkd2using TBMO. N represents the number of independent experiments. A pool of 10 animal caps was analyzed per experiment and treatment. The results from reporter mRNA alone served as reference and were set to 100% RLU. Relative values of single experiments are depicted as blue dots. Data of three experiments are presented as mean value (bar) ±standard deviation (error bar, SD). Statistical analyses were done with a one-sided Student’sttest for two independent means (Bonferroni corrected) using the values of three individual experiments.pvalues, values for individual experiments, mean values, and standard deviations are found in the source data file. n.s. not significant,p< 0.05; ** highly significantp< 0.01; ***, very highly significantp< 0.001, RLU relative luciferase units,Lucluciferase. 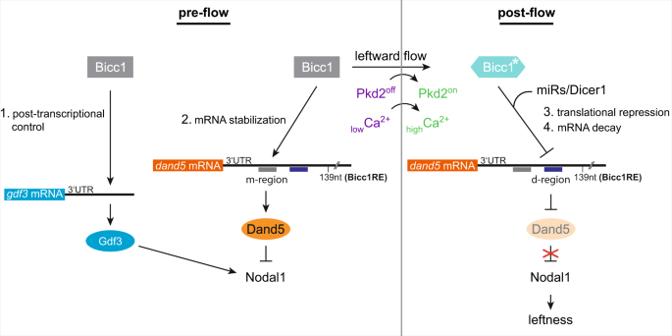Fig. 8: Two modes of Bicc1-dependent post-transcriptional regulation ofgdf3anddand5in flow sensor cells at theXenopusleft-right organizer. In the early neurula pre-flow stages, Bicc1 has two functions. Bicc1 assuresgdf3mRNA translation and thereby indirectly ensuresnodal1transcription by Gdf3 signaling. Simultaneously Bicc1 mediatesdand5mRNA stability via the medial (m) sub-region of the Bicc1RE. Thus, Dand5 protein levels are sustained on both sides, keeping Nodal in tight repression. Leftward flow activates the Pkd2 channel in left flow sensor cells, resulting in an asymmetric calcium signal. In post-flow stages, a calcium-dependent mechanism activates/modifies Bicc1 to become a repressor ofdand5translation, which is relayed by the distal (d) sub-region of the Bicc1RE. Subsequently,dand5mRNA gets degraded in a Dicer1 (miR) dependent manner. Attenuated Dand5 expression lifts repression of Nodal and defines leftness by induction of the LPM Nodal signaling cascade. For details, see text. Reporting summary Further information on research design is available in the Nature Research Reporting Summary linked to this article.